Substrate–water exchange in photosystem II is arrested before dioxygen formation Light-driven oxidation of water into dioxygen, catalysed by the oxygen-evolving complex (OEC) in photosystem II, is essential for life on Earth and provides the blueprint for devices for producing fuel from sunlight. Although the structure of the OEC is known at atomic level for its dark-stable state, the mechanism by which water is oxidized remains unsettled. Important mechanistic information was gained in the past two decades by mass spectrometric studies of the H 2 18 O/H 2 16 O substrate–water exchange in the four (semi) stable redox states of the OEC. However, until now such data were not attainable in the transient states formed immediately before the O–O bond formation. Using modified photosystem II complexes displaying up to 40-fold slower O 2 production rates, we show here that in the transient state the substrate–water exchange is dramatically slowed as compared with the earlier S states. This further constrains the possible sites for substrate–water binding in photosystem II. Photosynthesis provides the driving force for most life on Earth by converting sunlight into chemical energy. Cyanobacteria, algae and higher plants couple two photosystems in series to exploit water as the electron and proton source for the synthesis of carbohydrates from CO 2 . In the process they replenish the atmosphere with the dioxygen we live on. The complex four-electron four-proton chemistry of water oxidation is catalysed in photosystem II (PSII) by an inorganic cluster containing the earth-abundant metals Mn and Ca, which are bridged by five oxygen [1] , [2] , [3] , [4] , [5] , [6] , [7] , [8] , [9] . The structure of this Mn 4 CaO 5 cluster, which together with its ligands forms the oxygen-evolving complex (OEC), is now known at the atomic scale in its dark-stable state [4] . Density functional theory-based refinements have provided OEC structures ( Fig. 1a ) that can rationalize the vast majority of the available spectroscopic data [6] , [7] , [8] , [10] , [11] , [12] , [13] , [14] . 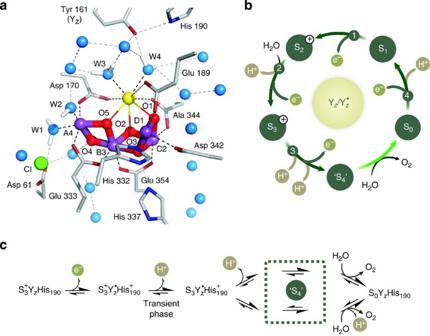Figure 1: The water-oxidizing complex in PSII and its reaction sequence. (a) Density functional theory-based model of the Mn4CaO5cluster in the ‘open cube’ (S2EPR multiline) configuration together with its water derived ligands W1–W412. The model is inserted into the 1.9-Å crystal structure of photosystem II4. MnIII/IV, purple; Ca2+, yellow; oxo-bridges, red; water–oxygens, blue; Cl−, green; amino acid backbones, grey; carboxy-oxygen, red; and His-nitrogen, dark blue. (b) Kok cycle for water oxidation in PSII including proton release to the bulk8,22(see alsoSupplementary Note 1) and water-binding events27,28. TheSistates (i=0, …, 4) denote the oxidation state of the Mn4CaO5cluster relative to theS0state, while the plus sign indicates a positive extra charge. (c) Detailed sequence of known and postulated states during molecular oxygen formation. Protons released in sequencecmay in part be taken up by internal bases created in earlierSistate transitions29. Figure 1: The water-oxidizing complex in PSII and its reaction sequence. ( a ) Density functional theory-based model of the Mn 4 CaO 5 cluster in the ‘open cube’ (S 2 EPR multiline) configuration together with its water derived ligands W1–W4 [12] . The model is inserted into the 1.9-Å crystal structure of photosystem II [4] . Mn III/IV , purple; Ca 2+ , yellow; oxo-bridges, red; water–oxygens, blue; Cl − , green; amino acid backbones, grey; carboxy-oxygen, red; and His-nitrogen, dark blue. ( b ) Kok cycle for water oxidation in PSII including proton release to the bulk [8] , [22] (see also Supplementary Note 1 ) and water-binding events [27] , [28] . The S i states ( i =0, …, 4) denote the oxidation state of the Mn 4 CaO 5 cluster relative to the S 0 state, while the plus sign indicates a positive extra charge. ( c ) Detailed sequence of known and postulated states during molecular oxygen formation. Protons released in sequence c may in part be taken up by internal bases created in earlier S i state transitions [29] . Full size image Water oxidation to dioxygen is energetically driven by light-induced charge separations within the reaction centre of PSII. These occur between the chlorophyll-containing photo-oxidant P680/ and the primary electron acceptor pheophytin. The OEC and P680 are connected via the redox-active tyrosine residue 161 of the D1 protein (Y Z / ) ( Fig. 1a ). In this way the OEC steps in response to short light flashes almost in synchrony through the four (semi)-stable oxidation states S 0 Y Z , S 1 Y Z , S 2 + Y Z and S 3 + Y Z ( Fig. 1b ), where the subscript signifies the number of stored oxidizing equivalents, and the plus sign indicates an extra charge caused by the lack of proton release during the transition from the dark-stable S 1 Y Z state to the S 2 + Y Z state. These (semi)-stable intermediates of water oxidation can be trapped with high yield and are thereby readily accessible for biophysical investigation. Although it is largely agreed that the S-state transitions between S 0 Y Z and S 3 + Y Z involve Mn-centred oxidation of the Mn 4 CaO 5 cluster [6] , [9] , [15] , some experimental results suggest ligand (oxo-bridge) participation and/or a structural change during the S 2 + Y Z ⇒ S 3 + Y Z transition [16] , [17] , [18] . The dark-stable S 1 Y Z state is generally considered to have the formal oxidation states Mn 4 (III,III,IV,IV) (high oxidation state scenario) [6] , [15] , [19] , but also the lower valent Mn 4 (II,III,III,IV)/Mn 4 (III,III,III,III) options are discussed [20] , [21] . Water oxidation starts only after the fourth oxidizing equivalent has been accumulated in the OEC, that is, once the transient state is reached ( Fig. 1c ). It is widely agreed that this dioxygen-forming reaction sequence starts with a proton release during the → transition [22] , [23] , [24] , [25] , followed by the formation of a Ca- or Mn-bound oxyl radical or of a Mn V -oxo group due to oxidation of the cluster by [6] , [14] , [26] . Although the following reaction steps towards O 2 must include the formation of a bound peroxidic intermediate, dioxygen formation and release, and the rebinding of substrate water [27] , [28] ( Fig. 1c ), the exact nature of the chemistry involved remains unsettled, as these transient states have so far largely eluded biophysical investigations [6] , [14] , [28] , [29] , [30] , [31] , [32] . O–O formation by nucleophilic attack may occur, for example, either between a free ( Fig. 2a ) [29] or a Ca-bound ( Fig. 2b ) [32] , [33] , [34] , [35] substrate water (the term ‘substrate water’ is used throughout the manuscript irrespective of the protonation state of the substrate oxygen) and a Mn V =O or Mn IV -oxyl radical. Alternatively, the O–O bond may be formed via radical coupling between either a Ca-oxyl radical and an Mn-bound oxyl radical ( Fig. 2c ) [14] , or between an Mn-oxyl radical and an Mn-oxo (bridge) ( Fig. 2d ) [6] , [30] , [31] , [36] . 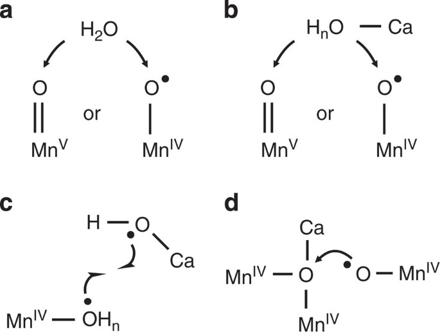Figure 2: Conceivable O–O bond formation mechanisms in the ‘S4’ state of PSII. (a) Nucleophilic attack by a bulk water onto a MnV=O or MnIV-oxyl radical29, (b) nucleophilic attack by a Ca bound water onto a MnV=O or MnIV-oxyl radical26,32,33,34,35, (c) coupling of a Ca-hydroxyl radical with a Mn-bound radical substrate14, (d) direct coupling between a terminal Mn-oxyl radical with an oxo bridge between Ca and Mn6,28,30,31,36. Figure 2: Conceivable O–O bond formation mechanisms in the ‘S 4 ’ state of PSII. ( a ) Nucleophilic attack by a bulk water onto a Mn V =O or Mn IV -oxyl radical [29] , ( b ) nucleophilic attack by a Ca bound water onto a Mn V =O or Mn IV -oxyl radical [26] , [32] , [33] , [34] , [35] , ( c ) coupling of a Ca-hydroxyl radical with a Mn-bound radical substrate [14] , ( d ) direct coupling between a terminal Mn-oxyl radical with an oxo bridge between Ca and Mn [6] , [28] , [30] , [31] , [36] . Full size image Substrate–water exchange experiments, which monitor the rate of incorporation of isotopically labelled bulk water into the substrate sites of the OEC, have allowed determining the relative binding characteristics of the two substrate–water molecules in all (meta)-stable S i Y Z states under various conditions, and have thereby provided unique insight into the mechanism of photosynthetic water oxidation [28] , [29] , [30] , [31] , [37] , [38] , [39] , [40] . In these experiments, PSII samples are preset to the desired S i Y Z state by light flashes, and are then rapidly mixed with H 2 18 O. After desired incubation times they are further advanced by flashes to produce dioxygen. The isotopic composition of the product O 2 ( 16,16 O 2 , 16,18 O 2 , 18,18 O 2 ) is monitored by membrane-inlet mass spectrometry [41] , and the substrate–water exchange rates are calculated from the H 2 18 O incubation time dependence of the m/z 34 and m/z 36 signals [26] , [42] . Assessing whether the two substrate waters can still exchange with the bulk water just before O–O bond formation, that is, in the transient and states, is expected to provide additional information on the nature and the binding sites of the two substrate waters, and therefore on the chemistry of water oxidation. Thus far, only very few time-resolved studies were able to probe these two transient states [22] , [24] , [25] , [43] , [44] and no information about substrate–water binding in the and states is available as yet. This is mainly because the halftimes of these states in native PSII samples are too short (≤1–2 ms) with respect to the mixing dead time in the water-exchange experiments ( t 1/2 =3 ms; see Supplementary Fig. 1 ). Recent studies set conditions though whereby the lifetimes of these transient states can be extended while preserving the overall function of the enzyme [45] , [46] . It was found that Thermosynechococcus elongatus cells growing on Sr 2+ -containing media devoid of Ca 2+ incorporate Sr 2+ in place of Ca 2+ into the OEC and that Cl − can be exchanged biochemically against Br − or I − ( Fig. 1a ); importantly, these substitutions have only minor structural effects [9] , [47] , [48] , [49] , [50] , but extend the half-lifetime of the state to 7 ms (Sr/Br-PSII) or even 45 ms (Sr/I-PSII) [45] , [46] . These samples thereby provide the opportunity to probe the rates of substrate–water exchange in this last transient before O 2 formation ( Fig. 1c ). Here we show that the exchange of both substrate waters is strongly retarded in the transient state as compared with the semi-stable S 3 + Y Z state. Four possible mechanisms for this simultaneous retardation of the exchange of both substrate waters induced by Y Z oxidation and the subsequent deprotonation of the catalytic site are presented and evaluated. On the basis of this evaluation and present literature data we conclude that W2 is most likely to be the fast exchanging substrate water (W f ), while O5 (or W3) can be assigned to be the slowly exchanging substrate water (W s ). Substrate–water exchange in the S 3 + Y Z state Substrate–water exchange measurements were performed for the S 3 + Y Z state to determine the influence of co-factor substitution on the substrate–water binding affinity in PSII core samples of T. elongatus . For this, the dark-adapted PSII samples were excited with two saturating flashes to advance the PSII complexes from the dark-stable S 1 Y Z state into the semi-stable S 3 + Y Z state. H 2 18 O was then injected at defined times before inducing dioxygen formation by giving one additional flash to the enzyme [26] , [28] , [37] . Figures 3a,b compare the substrate–water exchange kinetics in the S 3 + Y Z state of native Ca/Cl samples of T. elongatus with samples in which these cofactors were replaced by either Sr/Br or Sr/I. The native Ca/Cl-PSII shows the typical biphasic kinetics for the rise of the mixed labelled 16,18 O 2 ( Fig. 3a ), and the corresponding monophasic rise for the doubly labelled 18,18 O 2 species ( Fig. 3b ). As described previously, the fast 16,18 O 2 rise reflects the exchange of the fast exchanging substrate water (W f ), while the subsequent slow increase of the 16,18 O 2 signal and the rise of the double-labelled 18,18 O 2 species ( Fig. 3b ) reflect the exchange of the slowly exchanging substrate water (W s ) [26] . 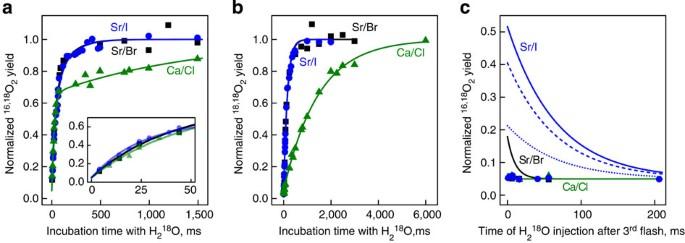Figure 3: Substrate–water exchange inT. elongatusPSII core particles containing different ionic cofactors. (a,b) The substrate water exchange in the S3+YZstate atm/z34 (16,18O2;a) andm/z36 (18,18O2;b), whilecdisplays the exchange in thestate atm/z=34. Symbols mark the data points (green triangles, Ca/Cl-PSII; black squares, Sr/Br-PSII; blue circles, Sr/I-PSII), while full lines are fits representing the fast and slow substrate–water exchange (a,b; for rate constants seeTable 1) or simulations of the expected experimental outcome assuming the exchange rates are identical in the S3+YZandstates (c). The blue dashed and dotted lines increpresent simulations where either the slow (dashed) or fast (dotted) rate of exchange was set to be 1,000 times slower than that measured in the S3+YZstate (Table 1). All data points (n=1) are normalized to values reached after complete isotopic equilibration. Each time course was measured once, but consists of many separately measured data points that were in part obtained on different days. Figure 3: Substrate–water exchange in T. elongatus PSII core particles containing different ionic cofactors. ( a , b ) The substrate water exchange in the S 3 + Y Z state at m/z 34 ( 16,18 O 2 ; a ) and m/z 36 ( 18,18 O 2 ; b ), while c displays the exchange in the state at m/z =34. Symbols mark the data points (green triangles, Ca/Cl-PSII; black squares, Sr/Br-PSII; blue circles, Sr/I-PSII), while full lines are fits representing the fast and slow substrate–water exchange ( a , b ; for rate constants see Table 1 ) or simulations of the expected experimental outcome assuming the exchange rates are identical in the S 3 + Y Z and states ( c ). The blue dashed and dotted lines in c represent simulations where either the slow (dashed) or fast (dotted) rate of exchange was set to be 1,000 times slower than that measured in the S 3 + Y Z state ( Table 1 ). All data points ( n =1) are normalized to values reached after complete isotopic equilibration. Each time course was measured once, but consists of many separately measured data points that were in part obtained on different days. Full size image The biological substitution of Ca 2+ by Sr 2+ leads to a tenfold acceleration of the slow exchange without significantly affecting W f ( Fig. 3a,b and Table 1 ). This is in good agreement with an earlier higher plant study, in which biochemical replacement of Ca 2+ by Sr 2+ was found to cause a fourfold acceleration of W s exchange [51] . This specific effect on the slow substrate–water exchange is useful, as it allows the detection of the exchange of both substrate waters in the state (see below). Finally, the substitution of Br − for I − has only a modest effect on the water exchange in the S 3 + Y Z state as evidenced by the similar exchange characteristics obtained with the Sr/Br- and Sr/I-PSII samples ( Fig. 3a,b ). Table 1 Rate constants of proton and electron transfer and water exchange during O 2 formation in PSII. Full size table Substrate–water exchange in the state On the basis of the exchange rates determined for the semi-stable S 3 + Y Z state, substrate water-exchange experiments in the transient state ( Fig. 3c ) were performed for all three sample types (Ca/Cl, Sr/Br, Sr/I). In these experiments, the dark-adapted PSII samples were advanced from the S 1 Y Z state by three saturating flashes into the transient state to initiate the O 2 -forming reaction sequence ( Fig. 1c ). After this third flash, H 2 18 O was injected at various delay times, and the 18 O incorporation into the product O 2 was monitored. The symbols in Fig. 3c show that no incorporation of the 18 O-label occurred for any of the three sample types, not even in the relatively long-lived state of the Sr/I-PSII samples. This shows that the bulk H 2 18 O exchanges too slowly with the already bound 16 O-substrate to allow incorporation of the 18 O-label into the O 2 product. The extent to which the substrate-water exchange is slowed in the state versus S 3 + Y Z is illustrated by the computed exchange curves in Fig. 3c . The longer lifetimes of both the and states should have resulted in relative 16,18 O 2 signals of 51(±6)% and 18(±2)% in the Sr/I-PSII and Sr/Br-PSII samples, respectively, if the exchange rates were the same as in the S 3 + Y Z state. Such yields are well above the detection limit, which allows the detection of 16,18 O 2 formation even at natural abundance ( Fig. 3c and Supplementary Fig. 2 ). Interestingly, the dashed and dotted blue curves show that a 1,000-fold slowing of only one of the exchange rates, while keeping the other one unchanged, cannot explain the data. Thus, our results imply that the exchange rates of both substrate waters are significantly retarded during the transitions. These simulations demonstrate that the corresponding other substrate water exchange rate needs to be additionally slowed by a factor >30 for W f (if W s is slowed by a factor of 1,000) and >10 for W s (if W f is slowed by a factor of 1,000), to make them consistent with the data. As a consequence, the exchange rate of W f in the state is<0.83 s −1 , and is thus at least tenfold slower than the exchange rate of W s in the S 3 + Y Z state of the Sr/I samples, and at least as slow as the exchange of W s in the Ca/Cl-PSII. It is emphasized that neither the overall oxygen production yield nor the period four oscillations were markedly affected by the cofactor substitutions [45] , [46] (see also Supplementary Fig. 3 ), showing that this observation is made with enzyme that despite the slowed final O 2 -producing transition functions normally. In catalysis, either in biology or in chemistry, isotope labelling studies are instrumental for elucidating reaction mechanisms [52] . In such experiments the substrate is labelled with a (stable) isotope and the propagation of this label into intermediates and/or the product(s) is followed. When studying the mechanism of water oxidation, H 2 18 O is typically added to a reactive species that has been pre-formed in unlabelled water. As an example, this method provided the demonstration that in a synthetic Mn-oxo complex, O 2 is produced by nucleophilic attack of hydroxide on Mn V ≡O (ref. 53 ). The characteristic signature for this mechanism is the evolution of 16,18 O 2 at a ratio equal to the 18 O-enrichment of bulk water. In contrast, we did not observe here any incorporation of 18 O into the dioxygen product above the natural abundance level, when injecting H 2 18 O into PSII suspensions poised in the state, even when the lifetime of the state was significantly lengthened by the exchange of Ca 2+ by Sr 2+ and Cl − by I − ( Fig. 3c ). It is noted that the state of PSII is comparable to Mn V in the above model complex in the sense that the O-O bond is formed without the acquisition of any additional oxidizing equivalents. In absence of an unprecedented diffusion barrier [54] , [55] , which would need to arise during the transitions, the observed lack of 16,18 O 2 formation directly excludes that in PSII the O–O bond is formed in the same way as in the Mn V ≡O model system [53] . In other terms, the nucleophilic attack of free water onto an electrophilic oxygen species ( Fig. 2a ) does not occur in PSII. This conclusion is consistent with previous data that showed that both substrate waters are bound to the OEC already in the S 2 and S 3 states [56] , [57] . However, nucleophilic attack of a Ca-bound water/hydroxo onto a group ( Fig. 2b ) [26] , [32] , [33] , [34] , [35] or coupling of a Ca-bound oxyl radical with a high valent Mn-oxo group ( Fig. 2c ) [14] may take place, if conditions are present in PSII that slow down the exchange of the Ca-bound substrate water seven to eight orders of magnitude over the exchange rates reported for water ligated to Ca 2+ in aqueous solutions [37] , [39] , [40] , [58] . Alternatively, both substrate –waters may be Mn-ligated and form the O–O bond via radical coupling ( Fig. 2d ) [6] , [30] , [31] , [36] . The lack of 16,18 O 2 and 18,18 O 2 production ( Fig. 3c ) demonstrates that the exchange of both substrate waters is significantly slower than the decay of the state into S 0 Y Z +O 2 , even when the O 2 production is severely slowed by cofactor exchange. The fact that the exchange of both substrate waters is slowed down so significantly despite a constant redox state of the Mn 4 CaO 5 cluster is important, and we discuss below the four possible mechanisms for ‘arresting’ both substrate waters under these conditions. The simplest possibility (mechanism 1) for slowing down significantly the exchange of both substrate waters would be the existence of the O–O bond (peroxide) already in the state [59] , [60] . At this point, the 18 O-label from the injected water could not be incorporated into the product and thus no 16,18 O 2 would be observed. Although internally consistent, this hypothesis is at odds with a recent time resolved X-ray spectroscopy experiment, which excluded Mn reduction (formation of the formal S 1 (O 2 ) 2− intermediate) during the transient phase ( Fig. 1c ). This implies that the O–O bond is formed at a later stage of the reaction cycle [8] , [43] , and rules out peroxide formation in the state as an explanation for the arrested water change. An alternative interpretation (mechanism 2) is that the oxidation state of Y Z strongly influences the substrate–water exchange via the H-bonding network around the Mn 4 CaO 5 cluster, which includes the two water ligands of Ca (W3 and W4; Fig. 1a ). The oxidation of Y Z (that is, formation) is coupled to the transfer of its phenolic proton to the nearby D1-His190 ( Fig. 1a ) [61] , [62] . This proton movement undoubtedly changes the H-bonding network [4] , [63] , [64] around the Y Z /Ca site and, as a consequence, may affect the exchange of the two substrate waters. This line of thought is partially supported by earlier data obtained with the alkaline-induced state (the dash denotes a likely difference in protonation state and/or water ligation with respect to the S 2 + Y Z state), which was generated by addition of base to the preformed S 3 + Y Z state [65] . These studies demonstrated that the substrate–water exchange is 5- to 20-fold slower in the state than in the S 2 + Y Z state [42] , [65] . The magnitude of this change is, however, too small to account for the 1000-fold decrease needed for at least one of the two substrates to explain the lack of 18 O-labelling of the dioxygen observed here ( Fig. 3c ). Nevertheless, this option cannot be completely ruled out, and, if true, would be a remarkable demonstration of the interconnectivity of all components of the OEC. A third option (mechanism 3) correlates the arrest of the substrate–water exchange with the deprotonation event on the Mn 4 CaO 5 (H n O) 4 cluster that was previously reported to occur during the transition ( Fig. 1c ) [22] and is demonstrated here to also occur in the Sr/Br-PSII samples ( Supplementary Figs 4–10 , Supplementary Note 1 and Supplementary Methods ). This proton release could explain a 1,000-fold decrease of one of the substrate–water exchange rates, if W f or W s is deprotonated. Notably, this could also account for a simultaneous slowing of the other substrate water (that is, at least 10- to 30-fold; see above), if the exchanges of both substrate waters are coupled (see ref. 28 ), or if the exchange of the other substrate is simultaneously slowed by mechanism 2. Finally (mechanism 4), a recent theoretical study concluded that substrate–water exchange can only occur in PSII, if at least one Mn ion within the Mn 4 CaO 5 cluster is in the Mn III redox state [40] . Thus, to exchange a water ligand in the S 3 + Y Z state, the Mn 4 CaO 5 cluster must first be transiently reduced by Y Z to generate the exchange-competent state (which may differ from the S 2 + Y Z and states discussed above in its protonation state and/or water binding). This requires the state and S 3 + Y Z state to be almost isoenergetic with low transition barrier, allowing for a fast redox equilibrium with an appreciable probability to form the state. If this is the mechanism for substrate exchange in the S 3 + Y Z state, then the substrate–water exchange in the state would indeed be expected to be impeded, simply because in this state the Mn 4 CaO 5 cluster cannot be transiently re-reduced by the oxidized . As such, our data provide the first experimental support to this theoretical prediction. We note, however, that mechanism 4 critically depends on the condition that both substrate waters are ligated to Mn and that all Mn ions in the S 3 + Y Z and states are in the oxidation state Mn IV , while the alternative explanations (mechanisms 2 and 3) do not. Experiments and theoretical calculations conducted by several groups have suggested that W2, W3, O5 ( Fig. 1a ) or WX (a water that is proposed to bind to the Mn 4 CaO 5 cluster during the S 2 + Y Z ⇒ S 3 + Y Z transition) are likely candidates for the two substrate waters [4] , [6] , [28] , [39] , [40] , [66] , [67] . In a very recent work, WX was ruled out as the immediate substrate by clearly demonstrating that both substrates are already bound in the S 2 + Y Z state [57] . Our present substrate–water exchange experiments in the S 3 + Y Z state ( Fig. 3a,b and Table 1 ) show that the exchange of W f is only marginally affected by biological Ca/Sr substitution, while the exchange of W s occurs ten times faster in the Sr-PSII sample. The fact that the difference between W f and W s is even stronger after biological substitution than after chemical exchange [51] considerably strengthens the previous suggestion [30] , [51] that W f is not a ligand of Ca 2+ . This point is further supported by the data presented here on water exchange in the state, which show that the exchange rate of W f is at least commensurate with the exchange rate of W s in the S 3 + Y Z state. Thus, from the short list above, W2 appears to be the most probable candidate for W f [39] , [57] . In contrast, the tenfold dependence of the binding affinity of W s on biosynthetic Ca/Sr substitution reported here provides additional strong support for a direct bond between Ca/Sr and W s [51] . This makes W3 (ref. 39 ) and O5 the most likely candidates for W s with O5 being favoured, owing to the S i Y Z state dependence of the W s exchange rate [28] , [30] , [58] , [67] even though a definitive assignment will require additional experimental support. For the first time, the exchangeability of the substrate–water molecules has been probed in the last transient state before the O–O bond formation. This provides important additional constraints for the ongoing identification of the substrate–water binding sites at the Mn 4 CaO 5 cluster and for the elucidation of the mechanism of water oxidation in PSII. The discovery that both substrate waters are non-exchangable in the last transient state before O 2 formation suggests that arresting the exchange of both substrate water molecules, rather than just one, is a mechanistic requirement. We propose, in line with the finding that the slowing down of oxygen evolution on Ca/Sr substitution stems from a change in entropy [68] , that this lack of exchange with the bulk water reflects a highly ordered arrangement of the OEC that is essential for low-energy O–O bond formation. Preparation of the PSII samples The T. elongatus strain used was the ΔpsbA1ΔpsbA2 deletion mutant [69] constructed from the T. elongatus 43-H strain that had a His6-tag on the carboxy terminus of CP43 (ref. 70 ). The biological Ca/Sr and the biochemical Cl/Br exchanges were achieved as previously described [45] , [46] , [68] . Ca/Cl-PSIIs, Sr/Cl-PSIIs and Sr/Br-PSIIs were purified with the protocol already described [68] . For the Cl − /I − exchange [46] , Sr/Cl-PSII’s bound to the Ni column were washed overnight with ~\n8–10 column volumes of a buffer containing 10% glycerol, 1 M betaine, 100 mM NaCl, 15 mM CaCl 2 , 15 mM, MgCl 2 , 40 mM MES, 1 mM L -histidine, 0.03% β-dodecyl maltoside, pH 6.5 (pH adjusted with NaOH). Next, the PSII core complexes bound to the resin were washed with one volume equivalent of a buffer containing 10% glycerol, 1 M betaine, 1 mM NaI, 15 mM Ca(OH) 2 , 15 mM Mg(OH) 2 , 1 mM L -histidine, 0.03% β-dodecyl maltoside, MES 40 mM, pH 6.5 (adjusted by addition of NaOH). The PSII’s were then eluted with a buffer containing, 1 M betaine, 1 mM NaI, 15 mM Ca(OH) 2 , 15 mM Mg(OH) 2 , 200 mM L -histidine, 0.03% β-dodecyl maltoside, pH 6.5 (adjusted by addition of MES powder). The eluted PSII samples were then washed by using Amincon-ultra-15 100 K concentrators in a buffer containing 1 M betaine, 1 mM NaI, 15 mM Ca(OH) 2 , 15 mM Mg(OH) 2 , 40 mM MES 40 mM, pH 6.5 (pH adjusted with NaOH). PSII samples were frozen at 77 K in liquid nitrogen until use. Substrate–water exchange measurements An isotope ratio mass spectrometer (ThermoFinnigan Delta plus XP) connected to a membrane-inlet cuvette (165 μl) via a cooling trap (liquid N 2 ) was used to measure substrate–water exchange at 20 °C [26] , [28] , [41] . The substrate–water exchange in the S 3 + Y Z state was studied by illuminating PSII, highly enriched in the state by a preflash and subsequent dark-adaptation, with two saturating Xe-flashes (2 Hz), followed by H 2 18 O injection at various times before the third flash, which was given at a fixed time after the second flash (6 s for Ca/Cl-PSII, 3 s for Sr/Br-PSII, 2 s for Sr/I-PSII). Four flashes (2 Hz) were given 5 min after the third turnover flash for normalization purpose. For the state measurements the -enriched PSII samples were illuminated with three flashes (2 Hz) followed by H 2 18 O injection at various times after the third flash, and the normalizing flash sequence. The S 3 + Y Z data were treated and fit within an Excel spread sheet employing equations 34 Y=0.66 (1−exp(− 34 k f •t))+0.34 (1−exp(− 34 k s •t)) and 36 Y=1−exp(− 36 k •t), where 34 Y and 36 Y signify the incubation time dependent 16,18 O 2 and 18,18 O 2 yields, respectively [26] , [42] . The expected 16,18 O 2 yields for the state experiments were calculated in 1 ms intervals and then summed up over the whole decay (3,000 ms) within Excel by folding the monoexponetial decay with the increasing H 2 18 O enrichment in the two binding sites. By varying the delay time between formation (third flash) and start of H 2 18 O enrichment (injection), the expected 16,18 O 2 yield was calculated for delays up to 210 ms. Injection artefacts, Chl dilution and H 2 18 O mixing were accounted for as in the S 3 + Y Z experiments. How to cite this article: Nilsson, H. et al. Substrate–water exchange in photosystem II is arrested before dioxygen formation. Nat. Commun. 5:4305 doi: 10.1038/ncomms5305 (2014).